High-resolution liquid patterns via three-dimensional droplet shape control Understanding liquid dynamics on surfaces can provide insight into nature’s design and enable fine manipulation capability in biological, manufacturing, microfluidic and thermal management applications. Of particular interest is the ability to control the shape of the droplet contact area on the surface, which is typically circular on a smooth homogeneous surface. Here, we show the ability to tailor various droplet contact area shapes ranging from squares, rectangles, hexagons, octagons, to dodecagons via the design of the structure or chemical heterogeneity on the surface. We simultaneously obtain the necessary physical insights to develop a universal model for the three-dimensional droplet shape by characterizing the droplet side and top profiles. Furthermore, arrays of droplets with controlled shapes and high spatial resolution can be achieved using this approach. This liquid-based patterning strategy promises low-cost fabrication of integrated circuits, conductive patterns and bio-microarrays for high-density information storage and miniaturized biochips and biosensors, among others. The interaction of liquids on surfaces is ubiquitous in our physical environment and also of importance to many areas of science and technology [1] , [2] , [3] , [4] , [5] , [6] , [7] , [8] . In nature, surface chemistry and roughness are widely used to manipulate liquid–solid interactions [9] , [10] . Inspired by these strategies, considerable efforts have focused on understanding, replicating and improving these approaches to design engineered fluidic-based systems [11] , [12] , [13] , [14] . A significant portion of research has been directed towards the design of efficient water-repellant surfaces, such as superhydrophobic surfaces, where droplets reside in a non-wetting composite state typically known as Cassie–Baxter droplets [15] . Cassie–Baxter droplets are desired for applications such as self-cleaning [12] , anti-icing [16] , drag reduction [17] , water harvesting [18] and condensation heat transfer [7] . Conversely, increasing roughness on hydrophilic surfaces is known to improve wetting (decrease the apparent contact angle), forming Wenzel droplets [19] , which are desired for applications where good solid–liquid contact is needed such as pesticide retention on plant surfaces [20] and boiling heat transfer [21] . Upon further increase in surface roughness, these Wenzel droplets eventually transition to thin-liquid films (via imbibition), which propagate due to enhanced capillarity generated by the surface roughness [22] . Such hydrophilic structured surfaces have accordingly been manipulated to perform interesting tasks, such as the formation of polygonal thin-liquid films [5] , uni-directional liquid spreading [6] and self-propagation of the liquid for thermal management and microfluidics applications [23] . Courbin et al . [5] demonstrated and qualitatively explained that liquids deposited on surfaces satisfying the imbibition condition can be manipulated to form square, hexagonal, octagonal and circular-shaped thin-liquid films. While this strategy provides excellent shape-selection ability [5] , [24] , the self-propagation of the liquid film on these surfaces presents practical challenges in using this strategy for applications that demand increased control and high spatial resolution. The ability to deposit desired liquid patterns with high accuracy and repeatability is particularly useful for liquid-based printing applications [25] , such as bio-microarrays for protein and DNA sequencing [26] , inkjet printing [27] , multicolour polymer-based light-emitting diode displays [28] , liquid metal printing [3] and solder droplet printing [2] . In this work, we show complete control of droplet contact area shapes ranging from squares, rectangles, hexagons, octagons, to dodecagons via the design of the structure or chemical heterogeneity on the surface. We use this versatile and robust strategy to demonstrate the ability to deposit high-density droplet arrays with complex wetting shapes on these simple-structured surfaces. In addition, the physical insights gained through the side and top-view visualization of the droplet dynamics aid in the development of a universal model for the three-dimensional droplet shape on microstructured surfaces. We believe that the understanding and the methodology developed in this work can be further tuned to deposit droplets with any predefined irregular shape, extending to even more diverse applications. Experimental methodology Well-defined cylindrical and cuboidal silicon micropillar arrays arranged in square, rectangular and hexagonal patterns were fabricated using standard contact photolithography and deep-reactive ion etching. Silane films were deposited on all samples such that the intrinsic contact angle (baseline contact angle on an equivalent smooth surface of the same chemical composition as the microstructured surface) could be controlled. Each sample was thoroughly cleaned before the start of the contact angle measurement experiment. A high-resolution microscopic contact angle meter (MCA-3, Kyowa Interface Science) was used to perform dynamic contact angle measurements on these microstructured samples. The details of the microfabrication, silanization, sample-cleaning procedure and contact angle measurement methodology are discussed in the Methods section. Droplet contact area and side-profile visualization Various droplet shapes and patterns obtained in this study are shown in Fig. 1 . 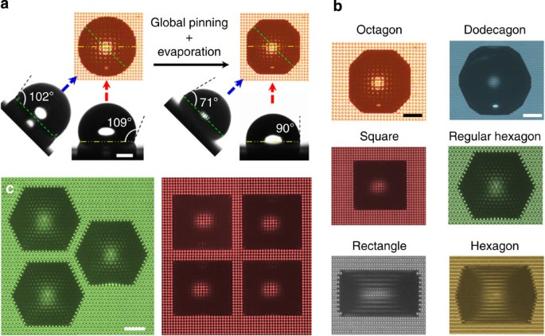Figure 1: False-colour images of various droplet shapes and patterns on micropillar surfaces. (a) Side- and top-view images of the droplet. The images on the left correspond to an advancing stage where the apparent contact angle is >90° and the actual contact line is not visible. The actual octagonal contact line is visible in the image on the right once the droplet evaporates in a global pinning mode and the apparent contact angle is <90°. The two side-view images acquired along the line-of-sight of 45° (second axes of symmetry, green dotted line) with respect to the pillar rows have been artificially rotated by 45°. The side-view images along with contact angles. (b) Different droplet shapes obtained by varying cylindrical micropillar array geometry. (c) The ability to pattern an array of microscopic droplets with excellent spatial control. Scale bar, 100 μm and the geometry is defined inSupplementary Table 1. The intrinsic contact angle (see Supplementary Table 1 for details of geometry and dimensions) was maintained below 90° (hydrophilic) by coating of these microstructured surfaces with phenyl-triethoxysilane and 3-(trimethoxysilyl) propyl methacrylate. Non-imbibing [22] Wenzel type droplets with spherical caps were formed where the apparent contact angle varied from ≈0° up to >90° ( Fig. 1a ). Attaining droplets with contact angles >90° on these intrinsically hydrophilic surfaces and the invalidity of the Wenzel equation [19] to predict this behaviour has been explained by local contact line pinning on the microstructure edges during the advancing stage [29] . We developed further insight into this process from detailed microscopic visualizations of the side and top profiles of deposited droplets on microstructured silicon surfaces ( Fig. 1a ). The images on the left correspond to an advancing stage where the apparent contact angle varies along the azimuthal direction. Since the apparent contact angle was uniformly >90°, the actual contact line was not visible until the droplet evaporated in a global pinning mode (everywhere along the contact line) such that the apparent contact angle along all directions was ≤90° (right). Figure 1: False-colour images of various droplet shapes and patterns on micropillar surfaces. ( a ) Side- and top-view images of the droplet. The images on the left correspond to an advancing stage where the apparent contact angle is >90° and the actual contact line is not visible. The actual octagonal contact line is visible in the image on the right once the droplet evaporates in a global pinning mode and the apparent contact angle is <90°. The two side-view images acquired along the line-of-sight of 45° (second axes of symmetry, green dotted line) with respect to the pillar rows have been artificially rotated by 45°. The side-view images along with contact angles. ( b ) Different droplet shapes obtained by varying cylindrical micropillar array geometry. ( c ) The ability to pattern an array of microscopic droplets with excellent spatial control. Scale bar, 100 μm and the geometry is defined in Supplementary Table 1 . Full size image The energy barriers associated with local contact line pinning were dependent on the spacing between the pillars and resulted in the loss of circular symmetry of the contact line on these surfaces. These insights inspired us to vary the microstructure geometry to realize a variety of other shapes (rectangles, stretched hexagons, stretched octagons and dodecagons) in addition to those (square, hexagon, octagon and circle) previously demonstrated via the thin-film mode (that is, during imbibition) of liquid shape formation on structured surfaces [5] ( Fig. 1b ). An octagonal droplet formed on a square array of cylindrical pillars, and upon increasing the pillar density ( D / L ) resulted in a square droplet. Similarly, a dodecagonal droplet formed on a hexagonal array of cylindrical pillars, and upon increasing the pillar density resulted in a hexagonal droplet. A square and a hexagonal droplet were converted to a rectangular and a stretched hexagonal droplet, respectively, by changing the pitch of these micropillars along one direction (see Supplementary Table 1 ; Fig. 1 ). Our approach also creates densely packed droplet arrays (≈40 μm spacing between droplets, Fig. 1c ) for liquid-based printing applications such as low-cost conductive patterns for integrated circuits, bio-microarrays for information storage and DNA and protein sequencing. Local contact line pinning at pillar edges High-resolution time-lapse images of the advancing microscopic contact line of a Wenzel droplet on a micropillar surface (diameter D =7 μm, pitch L =20 μm and height H =13 μm, Fig. 2a ) were obtained ( Fig. 2b ). The advancing ( θ F,A ) and the receding contact angles ( θ F,R ) on the corresponding flat surface coated with phenyl-triethoxysilane (Sigma-Aldrich) were 86° and 70°, respectively. Local contact line pinning at the pillar edges introduced a significant energy barrier for the advancing liquid front ( Fig. 2b ) to satisfy Gibb’s criteria [30] . The contact line that was locally pinned at the pillar top edge ( t =1 s), depins and advances by first wetting the sidewalls followed by the substrate base ( t =2 s). The local depinning results in an apparent decrease in the contact angle ( θ t= 1s > θ t= 2s ). The advancing contact line subsequently becomes pinned at the next row of pillars ( t =3 s) and the apparent contact angle continues to increase ( t =4 s) until it satisfies the local depinning criteria similar to that at t =1 s. As a result, despite the intrinsic hydrophilic (<90°) behaviour of the flat surface, the corresponding rough surface demonstrated an apparent hydrophobic behaviour where the advancing contact angles exceeded 90°. This observation contradicts the classical Wenzel equation, which predicts that the degree of hydrophilicity (hydrophobicity) of a surface increases upon increasing the roughness [19] . However, the Wenzel equation does not capture the advancing behaviour of these droplets since it does not account for the role of the local contact line pinning in the advancing stage ( Fig. 2c ). During a typical advancing stage, the portion of the contact line on the top surface of a micropillar ‘1’ advances with the local contact angle equal to the intrinsic contact angle on an equivalent flat surface ( θ F,A ). Once the advancing front approaches the pillar edge, the contact line becomes pinned ‘2’ and the local contact angle is required to exceed θ F,A +90°, ‘3’ for the front to advance further along the pillar sidewalls ‘4’. The high energy barrier associated with the local depinning contact angles of θ F,A +90° results in an apparent global pinning (everywhere along the contact line) and the unusually high advancing contact angle values on these otherwise hydrophilic ( θ F,A <90°) surfaces. 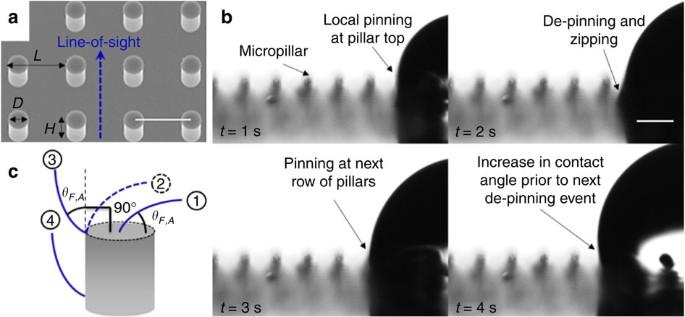Figure 2: Visualization of local contact line pinning. (a) A scanning electron micrograph (SEM) of a square array of cylindrical micropillar array with diameterD=7 μm, pitchL=20 μm and heightH=13 μm. (b) Time-lapse images of the local microscopic contact line dynamics of a Wenzel droplet. The line-of-sight for the acquisition of these images is shown ina. (c) Schematic illustrating the contact line dynamics that result in local energy barriers and contact line pinning responsible for the formation of wetting droplets with contact angles exceeding 90°. As a result, the classical Wenzel equation, which relies on global surface energy minimization, is invalid. Scale bar, 20 μm. Figure 2: Visualization of local contact line pinning. ( a ) A scanning electron micrograph (SEM) of a square array of cylindrical micropillar array with diameter D =7 μm, pitch L =20 μm and height H =13 μm. ( b ) Time-lapse images of the local microscopic contact line dynamics of a Wenzel droplet. The line-of-sight for the acquisition of these images is shown in a . ( c ) Schematic illustrating the contact line dynamics that result in local energy barriers and contact line pinning responsible for the formation of wetting droplets with contact angles exceeding 90°. As a result, the classical Wenzel equation, which relies on global surface energy minimization, is invalid. Scale bar, 20 μm. Full size image Estimation of advancing contact angle The contact angle of a growing Cassie–Baxter droplet θ CB,A on a chemically patterned surface with circular hydrophobic defects or on a superhydrophobic surface ( Fig. 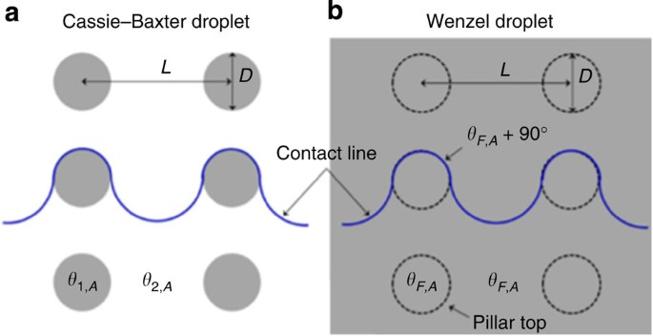Figure 3: Modelling of local contact line pinning. (a) Schematic of the advancing contact line movement via the Cassie–Baxter15mode on a chemically patterned surface. The background surface ‘2’ is relatively more wetting than the circular defects ‘1’, and hence, the contact line is distorted due to local pinning on ‘1’. (b) Similarly for the Wenzel19droplet on the right, the relatively large depinning contact angles at the pillar edges (θF,A+90°) result in local pinning and contact line distortion. 3a ) was previously [32] shown to be influenced by local contact line distortion and modelled as follows: Figure 3: Modelling of local contact line pinning. ( a ) Schematic of the advancing contact line movement via the Cassie–Baxter [15] mode on a chemically patterned surface. The background surface ‘2’ is relatively more wetting than the circular defects ‘1’, and hence, the contact line is distorted due to local pinning on ‘1’. ( b ) Similarly for the Wenzel [19] droplet on the right, the relatively large depinning contact angles at the pillar edges (θ F,A +90°) result in local pinning and contact line distortion. Full size image where θ 1,A and cos θ 2,A are the corresponding intrinsic advancing contact angles of the two background surfaces comprising the heterogeneous surface. Now, accounting for the contact line pinning at the pillar edges ( Fig. 2c ) on the surfaces investigated in this study where the local contact angle is required to exceed θ F,A +90° for the front to advance further along the pillar sidewalls ( Fig. 3b ), the apparent advancing contact angle of the Wenzel-type droplets in our study can be computed by replacing θ 1,A by θ F,A +90° and θ 2,A by θ F,A The subscript 0° indicates the direction of the line-of-sight for the side-view camera that, in this case, was parallel to the pillar rows ( Fig. 2a ). The experiment detailing the advancing, contact line pinning and receding modes of the droplet shown in Fig. 2 is also shown in Supplementary Movie 1 . The top- and side-profile visualization of the entire microscopic (diameter≈200 μm) droplet during the contact line pinning stage highlights an interesting asymmetry in the contact angles along the two principle axes of symmetry on the surface. The droplets in Fig. 4 were formed on a surface comprised of a square array of cylindrical micropillars with diameter D =7 μm, pitch L =20 μm and height H =13 μm. The images in Fig. 4a,b were acquired during two different but highly repeatable experiments, where the only difference was the line-of-sight for the side-profile visualization of the droplet. The side-profile images in Fig. 4a were captured such that the line-of-sight was parallel to the pillar rows (0° line-of-sight, first axes of symmetry) while the side-profile images in Fig. 4b were captured corresponding to a line-of-sight of 45° (second axes of symmetry) with respect to the pillar rows. Top-view images at t 1 right after the end of the advancing stage are shown on the top in Fig. 4a,b , as they could not be obtained during the advancing stage due to the obstruction from the piezo inkjet head used for liquid addition (see Supplementary Movie 2 ). Comparison of the corresponding side-profile images show an interesting anisotropy in the contact angle, where the apparent contact angle along the 45° line-of-sight ( θ A ,45° =102°, Fig. 4b at t 1 ) was smaller than that along the 0° line-of-sight ( θ A ,0° =109°, Fig. 4a at t 1 ). Despite the variation in depinning contact angles along the azimuthal direction during the advancing stage, the top images of the droplets appeared to preserve their spherical cap shape. The images in the bottom were acquired later at time t 2 when the droplet cap was shrinking in size during the global pinning stage, where the apparent contact angle continuously decreased to accommodate the mass loss by evaporation to the ambient. In particular, the images at time t 2 correspond to the case when the apparent contact angles along all directions were ≤90°, that is, the actual solid–liquid contact line was not masked and could be visualized in the top-view images. A comparison of the side profiles of the droplets also show asymmetry in the contact angle where, similar to t 1 , the apparent contact angle along the 45° line-of-sight ( θ 45° =71° in Fig. 4b at t 2 ) was smaller than that along the 0° line-of-sight ( θ 0° =90° in Fig. 4a at t 2 ). However, the droplet shapes deviated significantly from the typical spherical cap shape and an octagonal contact line is apparent in the top-view images. In spite of the continuous mass loss, the droplet base radius along the two axes of symmetry ( a 1 =199 μm, a 2 =210 μm,) did not change between t 1 and t 2 , that is, the shape of the droplet contact line was constant. The non-circular (octagonal) contact line just at the end of the advancing stage implies a non-circular advancing contact line during the liquid addition stage as well. 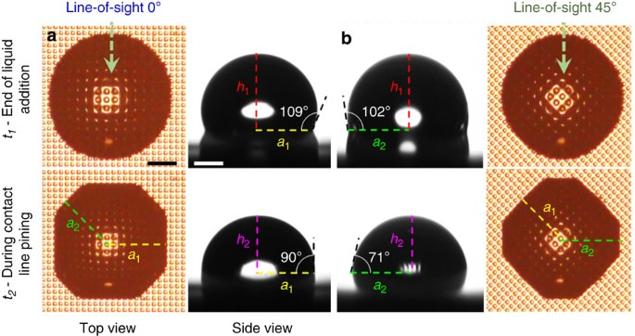Figure 4: Top- and side-profile visualization of a microscopic droplet. Images were captured during two different but highly repeatable experiments where the line-of-sight was (a) parallel and (b) at an angle of 45°with respect to the pillar rows. The top row of images (t1) correspond to the end of the advancing stage while the bottom row (t2) corresponds to an instant during the global pinning stage when the apparent contact angle along all directions was <90°. Scale bar, 100 μm. Figure 4: Top- and side-profile visualization of a microscopic droplet. Images were captured during two different but highly repeatable experiments where the line-of-sight was ( a ) parallel and ( b ) at an angle of 45 ° with respect to the pillar rows. The top row of images ( t 1 ) correspond to the end of the advancing stage while the bottom row ( t 2 ) corresponds to an instant during the global pinning stage when the apparent contact angle along all directions was <90 ° . Scale bar, 100 μm. Full size image The non-circular contact line shape is a result of the asymmetry in the depinning contact angles. We attribute this asymmetry in contact angles to the spacing between the pillars on a square array of cylindrical pillars, which changes from L along the 0° line-of-sight to along the 45° line-of-sight ( Fig. 5a ). The pillar density D / L , which is the critical parameter that dictates the depinning contact angles along the 0° line-of-sight, is modified to for contact angles measured along the 45° line-of-sight ( Fig. 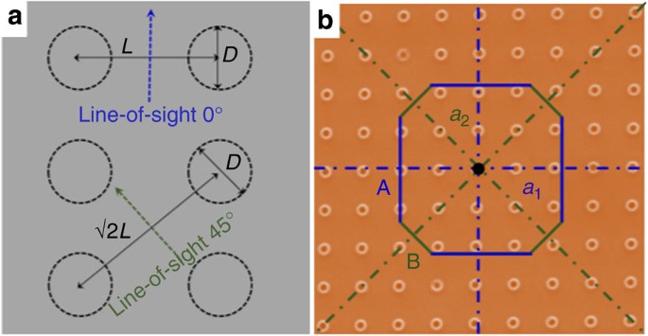Figure 5: Modelling of asymmetry in droplet shape. An illustration of the physical mechanism behind the anisotropy in depinning contact angles and hence the formation of an octagonal droplet on a square array of cylindrical pillars. (a) Pillar densityD/Lis the critical parameter that dictates the depinning contact angles along the 0° line-of-sight (parallel to the axes of symmetry). Accordingly, the ratio of diameterDto apparent pitchis the appropriate parameter governing the depinning contact angles along the 45° line-of-sight. (b) The apparent contact angles along these two directions are not the same, resulting in the loss of circular symmetry of the droplet contact area. Different depinning contact angles along the two directions but with the same droplet height implies unequal base radii along these directions. Since there are a total of four axes of symmetry, (two along the 0° line-of-sight and two along the 45° line-of-sight), an eight-sided polygon, that is, an octagonal contact line, is formed. 5a ) to yield: Figure 5: Modelling of asymmetry in droplet shape. An illustration of the physical mechanism behind the anisotropy in depinning contact angles and hence the formation of an octagonal droplet on a square array of cylindrical pillars. ( a ) Pillar density D / L is the critical parameter that dictates the depinning contact angles along the 0° line-of-sight (parallel to the axes of symmetry). Accordingly, the ratio of diameter D to apparent pitch is the appropriate parameter governing the depinning contact angles along the 45° line-of-sight. ( b ) The apparent contact angles along these two directions are not the same, resulting in the loss of circular symmetry of the droplet contact area. Different depinning contact angles along the two directions but with the same droplet height implies unequal base radii along these directions. Since there are a total of four axes of symmetry, (two along the 0° line-of-sight and two along the 45° line-of-sight), an eight-sided polygon, that is, an octagonal contact line, is formed. Full size image Since the advancing contact angles along the two line-of-sights described by equations (2) and (3) are different, the droplet contact line loses its circular symmetry. Unequal depinning contact angles along the two principle directions, but with the same droplet height ( h 1 , Fig. 4 ), implies unequal base radii along these directions ( a 1 ≠ a 2 ). Moreover, the presence of four axes of symmetry results in an octagonal contact line as shown in Fig. 5b . Experiments on 15 samples with various other micropillar geometries (see Supplementary Fig. 2a ) were performed to support the validity of equations (2) and (3). Good agreement between the model prediction and experimental depinning contact angles along both axes of symmetry ( Supplementary Fig. 2b,c ) was found. We also varied the pillar height to demonstrate the independence of the wetted shape, wetted area and advancing contact angle consistent with the predictions of equation (2) (height H was changed from ≈11–13 μm in Supplementary Fig. 2 to ≈20–23 μm in Supplementary Fig. 3 ). The surface chemistry was varied (phenyl-triethoxysilane coating that was used for validation in Supplementary Fig. 2 , and results in the intrinsic advancing contact angle θ F,A of 85°–89°, was replaced by 3-(trimethoxysilyl) propyl methacrylate coating such that the intrinsic advancing contact angle varied between 73° and 81° in Supplementary Fig. 4 ), which also showed good agreement between the experiments and model prediction, confirming the robustness of the model over a range of wetting parameters. Conversely, unlike the advancing stage, the micropillar surface did not provide local energy barriers during the receding phase, and the classical Wenzel equation [19] was found to be valid. The apparent receding contact angle of the droplet on rough and hydrophilic surfaces decreased with increasing roughness as follows: where cos θ R is the receding contact angle on the microstructured surface and θ F ,R is the intrinsic receding contact angle on an equivalent flat surface. This result is shown in Supplementary Fig. 5 where the same 15 samples previously tested for advancing contact angle in Supplementary Fig. 2 were investigated during the receding mode. The imbibition condition [22] was satisfied for samples 1, 2, 7, 10, 11 and 12. As a result, either a thin film or a receding droplet with near-zero contact angles was experimentally observed in these cases. Modelling of the contact area shape On the basis of our understanding of the reason droplets demonstrate dissimilar contact angles along different directions (line-of-sight), we developed a geometric model to predict the side-length ratio [31] B / A of the octagonal droplets in our experiments. Different depinning contact angles along the two directions, but with the same droplet height ( Fig. 4 ), implies unequal base radii ( a 1 ≠ a 2 ) along these directions. Using a simple geometric argument, the base radii along the two line-of-sights can be related to the respective depinning contact angles as follows: Unequal base radii along these directions implies unequal sides A and B (defined in Fig. 5b ) for the octagon. Further geometric manipulation yields: where θ A ,0° and θ A ,45° are given by equations (2) and (3), respectively. Since there are a total of four axes of symmetry ( Fig. 5b ), (two along the 0° line-of-sight and two along the 45° line-of-sight), an eight-sided polygon, that is, an octagonal contact line, is formed. Equation (6) also suggests that a regular octagon B / A ≈1 (an octagon with all sides equal), should be formed on low-density pillars, while a square droplet where B / A→ 0, can be formed by fabricating high-pillar density microstructured surfaces. This behaviour was observed in our experiments where octagonal droplets were formed on a low-density ( D / L =0.35) micropillar array, while liquid deposition on a high-density micropillar array ( D / L =0.7) resulted in the formation of square droplets ( Fig. 6a ). The agreement between the experimental results (black dots) and model prediction (black solid curve, equation (6)) supports the simple geometric model (equations (2) and (3)) discussed in Fig. 5 . The relative insensitivity of B / A to the intrinsic wettability ( θ F,A was varied from 45° to 87°) of these surfaces suggests that this approach is robust to create these shapes, where the deterioration in the surface coating, that is, the change in intrinsic contact angle, does not adversely affect the shape of the droplet that can be deposited on these surfaces. 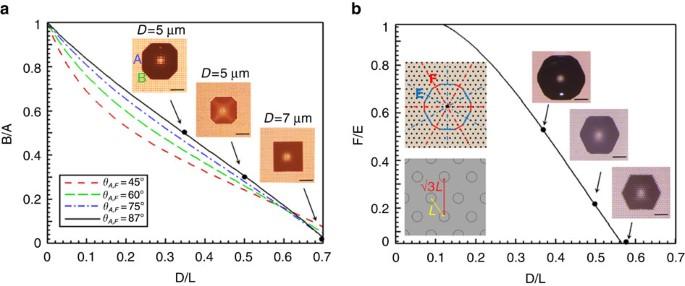Figure 6: Droplet shape transformations with changing micropillar geometry. (a) Comparison between experimental and model prediction of the ratio of octagon side lengths (B/A) versus pillar densityD/Lon square arrays of cylindrical micropillars. The ratio of octagon side length decreased with pillar density resulting in the formation of a square droplet whenD/L=0.7 for the intrinsic advancing contact angleθF,Aof 87°. (b) Comparison between experimental and model prediction of the ratio of dodecagon side lengths (F/E) versus pillar densityD/Lon hexagonal array of cylindrical micropillars. A hexagonal droplet was formed as the pillar density was increased. The intrinsic advancing contact angleθF,Aon an equivalent flat surface was 87°. Scale bar, 100 μm. Figure 6: Droplet shape transformations with changing micropillar geometry. ( a ) Comparison between experimental and model prediction of the ratio of octagon side lengths ( B / A ) versus pillar density D / L on square arrays of cylindrical micropillars. The ratio of octagon side length decreased with pillar density resulting in the formation of a square droplet when D / L =0.7 for the intrinsic advancing contact angle θ F,A of 87°. ( b ) Comparison between experimental and model prediction of the ratio of dodecagon side lengths ( F / E ) versus pillar density D / L on hexagonal array of cylindrical micropillars. A hexagonal droplet was formed as the pillar density was increased. The intrinsic advancing contact angle θ F,A on an equivalent flat surface was 87°. Scale bar, 100 μm. Full size image We extended the same principle to develop design guidelines for depositing droplets on hexagonal arrays. A hexagonal array of pillars also has two principles axes of symmetry, the first one parallel to the row of pillars with defined pitch L and the second one at an angle of 30°, where the apparent pitch is ( Fig. 6b ). Moreover, there are three such axes of symmetry of both types between 0° and 360°. As a result, a dodecagonal (polygon with 12 sides) droplet was formed on these surfaces. Similarly, a simple geometrical model was developed to predict the ratio of dodecagon side lengths ( F / E ), and showed excellent agreement with experimental droplet shapes shown in Fig. 6b . Analogous to the case of a square array of pillars where an octagon with the four axes of symmetry turned into a square upon increasing the pillar density, on a hexagonal array of pillars, a dodecagonal droplet turned into a hexagonal droplet upon increasing the pillar density. While the ability to deposit droplets of desired shapes in a highly repeatable manner is desired for high spatial-resolution liquid-based printing technologies, it can also be utilized to perform interesting tasks such as bi-directional liquid spreading for microfluidic applications. This concept is demonstrated in Fig. 7 , where the pitch between pillars along the x ( L ) and y ( M ) directions were changed, that is, the pitch along the y axis of a square array of cylindrical pillars was increased to form a rectangular array of circular pillars. Different pitches along the x ( L ) and y ( M ) directions implied different depinning contact angles along these two directions, resulting in elongated droplets. A droplet with a square wetted area that was formed on a high-density square array of a micropillar surface (diameter D =9 μm, pitch L =12 μm and height H =20 μm) was converted to a rectangular droplet upon increasing the pitch along the y axis, M>L , and forming a rectangular array of cylindrical micropillars (diameter D =9 μm, pitch along x , that is, L =12 μm, pitch along y , that is, M =22 μm and height H =20 μm). Interestingly, the elongation of the droplet was orthogonal (dotted arrow) to the direction along which the pitch was increased (solid arrow). If the pitch along the y axis was enlarged, a rectangle was formed where the side length along x was larger than that along y . The same strategy when applied to a hexagonal array of cylinders converted a hexagonal droplet to an elongated hexagonal droplet as shown in Fig. 7b . 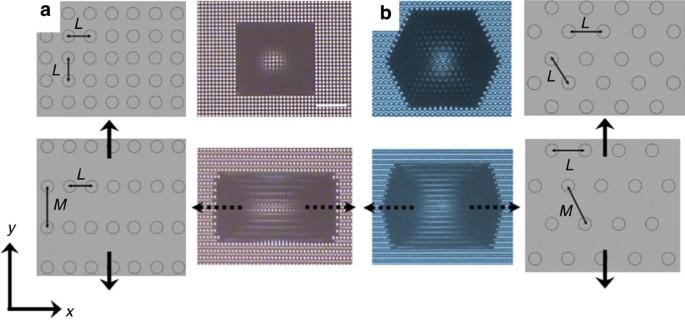Figure 7: Design strategy to stretch droplet shapes. (a) A droplet with a square wetted area formed on a high-density square array of a cylindrical micropillars was converted to a rectangular droplet upon increasing the pitch along one axis. Different pitches along thex(L) andy(M) directions implied different depinning contact angles along these two directions resulting in elongated droplets. (b) The same principle when applied to a regular hexagonal array of cylindrical micropillars resulted in a stretched hexagon orthogonal to the direction along which the pitch was increased. This strategy can be utilized to design surfaces with anisotropic liquid supply rates. Scale bar, 100 μm. Figure 7: Design strategy to stretch droplet shapes. ( a ) A droplet with a square wetted area formed on a high-density square array of a cylindrical micropillars was converted to a rectangular droplet upon increasing the pitch along one axis. Different pitches along the x ( L ) and y ( M ) directions implied different depinning contact angles along these two directions resulting in elongated droplets. ( b ) The same principle when applied to a regular hexagonal array of cylindrical micropillars resulted in a stretched hexagon orthogonal to the direction along which the pitch was increased. This strategy can be utilized to design surfaces with anisotropic liquid supply rates. Scale bar, 100 μm. Full size image It should be noted that the actual contact line shape during the advancing stage in many of these experiments were masked by the droplets when the apparent advancing contact angle values were >90°. For example, the rectangular contact line of a droplet on a rectangular array of cylindrical micropillars with the difference in the advancing contact angles along the y and x directions as high as 26° ( Fig. 8a , top) was only visible when the contact angles along both directions uniformly decreased below 90° due to evaporation to the ambient during the pinning mode ( Fig. 8a , bottom). This level of asymmetry for a liquid droplet is only possible due to the high energy barriers associated with localized pinning of the contact line along the pillar edges. 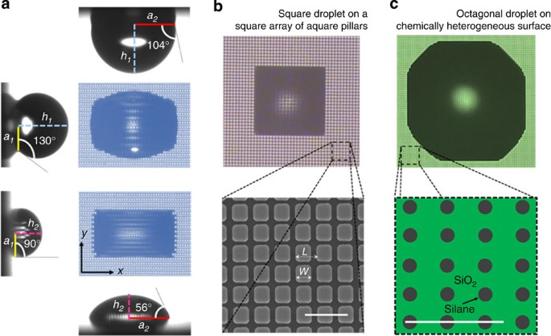Figure 8: Demonstration of the anisotropic droplet shape on different types of surfaces. (a) The difference in the advancing contact angles along theyandxdirections for a rectangular droplet were as high as 26° (top), which continued to increase further (bottom) as the droplet was pinned and the contact angle decreased during evaporation to ambient. This level of asymmetry in a liquid droplet is only possible due to the high energy barriers associated with the localized pinning of the contact line along the pillar edges. The strategy was further tested on other geometries: (b) cuboidal pillars and (c) chemically patterned and optically smooth surfaces (D=3 μm andL=8 μm). Scale bar, 20 μm. Figure 8: Demonstration of the anisotropic droplet shape on different types of surfaces. ( a ) The difference in the advancing contact angles along the y and x directions for a rectangular droplet were as high as 26° (top), which continued to increase further (bottom) as the droplet was pinned and the contact angle decreased during evaporation to ambient. This level of asymmetry in a liquid droplet is only possible due to the high energy barriers associated with the localized pinning of the contact line along the pillar edges. The strategy was further tested on other geometries: ( b ) cuboidal pillars and ( c ) chemically patterned and optically smooth surfaces ( D =3 μm and L =8 μm). Scale bar, 20 μm. Full size image The robustness of the approach to obtain different shapes was validated by changing the pillar shape ( Fig. 8b ), as well as on chemically patterned surfaces used in our previous work [32] ( Fig. 8c ). Images in Fig. 8b highlight the fact that the same understanding can be utilized to form droplets of different shapes with other pillar geometries. For an array of cuboidal pillars, the pillar density, that is, the ratio of pillar width W to the pitch L , is the critical parameter governing the shapes. Hence for the same value of D / L for cylindrical pillars and W / L for the cuboidal pillars, the same droplet shapes were obtained. The image in Fig. 8c (top) demonstrates the ability to obtain anisotropic droplets during the advancing phase on an optically smooth chemically patterned surface as well (square array of circular hydrophobic silane defects on a silica surface [32] , bottom). Similar shapes in the thin-film regime have been previously demonstrated [31] on chemically patterned surfaces as well, however, the droplets in our work are in the non-propagating regime with finite contact angles, allowing superior control than those with the self-propagating thin-liquid-film regime [5] . We have demonstrated the ability to deposit high-density droplet arrays with complex wetting shapes on a simple-structured surface. This versatile and robust strategy to form high-resolution liquid patterns via three-dimensional droplet shape control in a highly repeatable manner along with the detailed understanding of the physical mechanism behind these shapes promise advancements in liquid-based deposition and printing technologies. This work may be readily extended to a number of surface materials for specific applications by using a number of scalable manufacturing processes including, hot embossing, moudling and roll-to-roll. Furthermore, we believe that the methodology provided by this work can be tuned to deposit droplets with any predefined irregular shape as well, extending to diverse applications such as integrated circuits and conductive patterns, miniaturized biochips and biosensors, bio-microarrays, among many others. Test sample fabrication and coating Standard contact photolithography and deep-reactive ion etching were used to create silicon micropillar arrays. The scanning electron microscope images and the corresponding dimensions of the six representative test samples are shown in Supplementary Fig. 1 . The intrinsic contact angle of the surfaces was maintained <90° (hydrophilic) by depositing the microstructured surfaces with phenyl-triethoxysilane and 3-(trimethoxysilyl) propyl methacrylate (Sigma-Aldrich) using chemical vapour deposition. Before the start of the contact angle measurement experiment, all samples were rinsed with acetone and iso-propyl alcohol (Macron Chemicals, CAS no. 67-64-1 and 67-63-0, respectively) followed by deionized water and blow drying with N 2 . Contact angle experiments Dynamic contact angle measurements were performed at room temperature (22–25 °C) and a relative humidity of 40–65%. An automatic microscopic contact angle meter (MCA-3, Kyowa Interface Science) was used for the experiments. Reagent grade water (Sigma-Aldrich, CAS no. 7732-18-5) was used as the fluid. A piezo inkjet (PIJ) head dispensed ultrasmall droplets with a volume of ≈20 picolitres at a rate of 100 Hz (2.0 nl s −1 ) for 15 s allowing ample time to monitor the advancing contact angle. The PIJ was then turned off and the droplet was monitored while evaporating. Absence of any observable residue after complete droplet evaporation ruled out contamination effects from the test fluid. Liquid addition rates were varied from 0.15 nl s −1 at 10 Hz to 3.0 nl s −1 at 200 Hz to confirm the negligible influence of the PIJ-dispensing frequency on contact angle behaviour. Side and top droplet profiles were acquired at 1 and 30 Hz, respectively. Owing to the placement of the PIJ during the droplet-advancing phase, top-view images could only be acquired during evaporation (pinning and receding phases). Image analysis Embedded image processing software used the half-angle method to determine the contact angle with a high resolution of 0.1° from the side-view images. The half-angle method assumes a spherical cap and calculates the contact angle θ from the angle φ between the droplet baseline and the line passing beyond the apex of the droplet (which is a valid assumption for a maximum droplet volume ≈25 nl). The contact angles were repeatable to within ±2° and the uncertainty in measurements was within ±1°. How to cite this article: Raj, R. et al . High-resolution liquid patterns via three-dimensional droplet shape control. Nat. Commun. 5:4975 doi: 10.1038/ncomms5975 (2014).